Phosphorylation of VE-cadherin is modulated by haemodynamic forces and contributes to the regulation of vascular permeabilityin vivo Endothelial adherens junctions maintain vascular integrity. Arteries and veins differ in their permeability but whether organization and strength of their adherens junctions vary has not been demonstrated in vivo . Here we report that vascular endothelial cadherin, an endothelial specific adhesion protein located at adherens junctions, is phosphorylated in Y658 and Y685 in vivo in veins but not in arteries under resting conditions. This difference is due to shear stress-induced junctional Src activation in veins. Phosphorylated vascular endothelial-cadherin is internalized and ubiquitinated in response to permeability-increasing agents such as bradykinin and histamine. Inhibition of Src blocks vascular endothelial cadherin phosphorylation and bradykinin-induced permeability. Point mutation of Y658F and Y685F prevents vascular endothelial cadherin internalization, ubiquitination and an increase in permeability by bradykinin in vitro . Thus, phosphorylation of vascular endothelial cadherin contributes to a dynamic state of adherens junctions, but is not sufficient to increase vascular permeability in the absence of inflammatory agents. The control of vascular permeability is of pivotal importance in several vascular pathologies including inflammation, interstitial oedema, ischaemic stroke and others [1] , [2] , [3] . Besides transcellular transport systems, plasma fluids can cross the endothelial barrier through cell junctions. These specialized structures include tight and adherens junctions (AJ), which maintain endothelial cell-to-cell adhesion [2] , [4] , [5] . At endothelial AJ, adhesion is mediated by a cell-specific member of the cadherin protein family called vascular endothelial cadherin (VEC) [2] , [6] , [7] . VEC promotes homophilic adhesion and forms zipper-like structures along endothelial cell contacts. The cytoplasmic domain of VEC interacts with several intracellular partners, including β-catenin, plakoglobin and p120, which transfer intracellular signals and modulate interaction with the actin cytoskeleton [2] , [6] , [7] . VEC has an important role in the control of vascular permeability in vitro and in vivo [1] , [2] , [3] , [7] , [8] , [9] , [10] , [11] , [12] . Blocking antibodies to VEC induce a dramatic increase in lung and heart permeability accompanied by oedema and hemorrhages [8] . More subtle changes in the organization and strength of AJ are associated with tyrosine phosphorylation of the VEC cytoplasmic domain in cultured cells or organ extracts [11] , [13] , [14] . Much of our knowledge of the molecular regulation of permeability is based on cultured endothelial cells. Although informative, in vitro systems do not fully reproduce in vivo conditions. Most importantly, different types of vessels respond quite differently to inflammatory mediators in vivo . For instance, veins are the typical targets of inflammatory mediators while small-calibre arteries are rarely affected [1] , [15] . This suggests that there are mechanisms that sensitize veins to inflammatory mediators in vivo . In the present study, we approached this issue using specific antibodies against phosphorylated VEC. Surprisingly, we found that in vivo VEC is constitutively tyrosine phosphorylated in veins but not in arteries. VEC phosphorylation is likely mediated by mechanosensor mechanism(s) that activate junctional Src under venous shear stress. Src inhibitors block VEC phosphorylation and bradykinin-induced vascular permeability. In searching for a mechanism of action we found that phosphorylation makes VEC particularly sensitive to bradykinin-induced endocytosis which, in turn, mediates a rapid but reversible increase in vascular permeability. Although VEC internalization has been reported to be a crucial step in the increase of vascular permeability in vitro [4] , [10] , this report is the first to monitor modifications of endothelial junction architecture in vivo under normal and pathological conditions. Development of antibodies against phosphorylated VEC In order to test the relevance of tyrosine phosphorylation of VEC (pYVEC) in vivo , we developed two antibodies directed against phospho-peptides of the cytoplasmic region of VEC corresponding to amino acid 646–669 (spanning Y658; antibody pY658-VEC) and to amino acid 671–700 (spanning Y685; antibody pY685-VEC) ( Fig. 1 ). We selected these two peptidic sequences as they were predicted to be strongly antigenic, the respective tyrosines are highly conserved among species and were previously found to be phosphorylated by permeability-increasing agents [12] , [16] , [17] . Furthermore, phosphorylation of Y658 was reported to reduce the binding of p120, an important stabilizer of cadherins at the cell membrane [18] , [19] . Y685 is a target of Src [12] and its phosphorylation modulates the association of the kinase csk, an inhibitor of src and implicated in contact inhibition of cell growth [16] . The antibodies were affinity-purified against the respective antigen and absorbed on VEC-null endothelial cells for any residual non-specific binding. Specificity was further supported through multiple in vitro and in vivo tests. First, the two antibodies did not recognize VEC in which the region of amino acid 622–702 ( Fig. 1b ), spanning both phosphopeptides ( Fig. 1a ), was deleted [20] . The same mutant was instead recognized by the commercially available pY658-antibody ( Fig. 1h ). Second, both antibodies codistributed with an anti total-VEC antibody but did not recognize endothelial cells treated with VEC short interfering RNA (siRNA) ( Fig. 1c ), VEC-null endothelial cells [20] ( Fig. 1d ) or VEC null embryos [21] ( Supplementary Fig. S1a ). Third, in pervanadate-treated cells, point mutation in phenylalanine (Y658F and Y685F) abolished both staining and recognition by western blot of the respective antibody ( Fig. 1e–g ). Conversely, both antibodies recognized VEC-wild-type (wt) or the unrelated mutant ( Fig. 1e–g ). Pixels of VEC/pYVEC co-localization are highlighted in white in Fig. 1e (right panel) (pY658-VEC) and Fig. 1f (right panel) (pY685-VEC). Fourth, both antibodies gave a junctional specific in vivo staining ( Fig. 2 ), which was inhibited by coincubation with the respective phospho-peptides, but not with the corresponding non-phospho-peptides ( Supplementary Fig. S1b ). The pY685-VEC antibody was effective in binding mouse VEC but weak on human VEC because of low homology of the peptide antigen ( Fig. 1a ). By contrast, antibody pY658-VEC could bind VEC in both species. Therefore, the experiments performed on human umbilical vein endothelial cells (HUVEC) were done with antibody pY658-VEC. Staining of murine VEC (mVEC) with either pY658 or pY685 appears to give comparable results (see below). In this work we studied phosphorylation of Y658 and Y685 only and along the text we refer to pYVEC when the protein is recognized by the two anti-pY658-VEC and pY685-VEC antibodies. 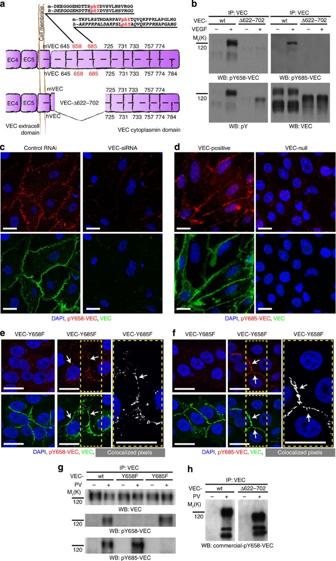Figure 1: pY658- and pY685-VEC antibodies specifically recognize phosphorylated VEC in vitro. (a) The cytoplasmic tail of murine VEC and human VEC contains eight and nine tyrosine residues, respectively, as indicated. Antibodies to murine pYVEC have been developed using the sequences around residue Y658 and Y685 (red), respectively. The corresponding human (hVEC) sequences are reported. The sequence deleted in human VEC-Δ622-702 mutant is indicated. (b) Immunoprecipitation (IP) of wt human VEC followed by western blot (WB) showed that antigen recognition by pY658-VEC and pY685-VEC antibodies was increased upon 5 min VEGF treatment. Both pYVEC antibodies did not recognize the VEC-Δ622-702 mutant, conversely an unselective anti-phosphorylated tyrosine antibody (pY) could bind both VEC-wt and VEC-Δ622-702 mutant. (c) VEC-siRNA treatment of VEGF-stimulated HUVEC inhibited pY658-VEC staining (in red) of endothelial cells junctions, VEC is shown in green. Scale bar: 20 μm. (d) Antibody pY685-VEC did not decorate cell junctions of VEGF-stimulated mVEC-null endothelial cells (right panels). Staining with pY658-VEC gave comparable results (not shown). Scale bar: 20 μm. (e) Antibody pY658-VEC did not bind to VEC-Y658F mutant (left panels), but recognized VEC-Y685F mutant (central and right panels) in pervanadate-treated cells. (f) Conversely, antibody pY685-VEC did not recognize VEC-Y685F mutant (left panels) but could bind to VEC-Y658F mutant (central and right panels) in pervanadate treated cells. Pixels presenting the co-localization of pY658- or pY685-VEC with total VEC are highlited in white. Scale bar: 50 μm. (g) Antibody pY658-VEC did not bind to immunoprecipitated VEC-Y658F mutant (central lanes), but recognized VEC-wt or VEC-Y685F mutant (left and right lanes). Conversely, antibody pY685-VEC did not recognize immunoprecipitated VEC-Y685F mutant (right lanes), but could bind to VEC-wt or VEC-Y658F mutant in pervanadate-treated cells (left and central lanes). (h) IP of wt hVEC followed by WB showed that antigen recognition by the commercially available antityrosine-phosphorylated-(Y658)-VEC antibody was increased upon pervanadate treatment. However, the antibody tested was also equally able to recognize the VEC-Δ622-702 mutant, in which the indicated tyrosine is not present. Data shown are representative of at least three independent experiments. Figure 1: pY658- and pY685-VEC antibodies specifically recognize phosphorylated VEC in vitro. ( a ) The cytoplasmic tail of murine VEC and human VEC contains eight and nine tyrosine residues, respectively, as indicated. Antibodies to murine pYVEC have been developed using the sequences around residue Y658 and Y685 (red), respectively. The corresponding human (hVEC) sequences are reported. The sequence deleted in human VEC-Δ622-702 mutant is indicated. ( b ) Immunoprecipitation (IP) of wt human VEC followed by western blot (WB) showed that antigen recognition by pY658-VEC and pY685-VEC antibodies was increased upon 5 min VEGF treatment. Both pYVEC antibodies did not recognize the VEC-Δ622-702 mutant, conversely an unselective anti-phosphorylated tyrosine antibody (pY) could bind both VEC-wt and VEC-Δ622-702 mutant. ( c ) VEC-siRNA treatment of VEGF-stimulated HUVEC inhibited pY658-VEC staining (in red) of endothelial cells junctions, VEC is shown in green. Scale bar: 20 μm. ( d ) Antibody pY685-VEC did not decorate cell junctions of VEGF-stimulated mVEC-null endothelial cells (right panels). Staining with pY658-VEC gave comparable results (not shown). Scale bar: 20 μm. ( e ) Antibody pY658-VEC did not bind to VEC-Y658F mutant (left panels), but recognized VEC-Y685F mutant (central and right panels) in pervanadate-treated cells. ( f ) Conversely, antibody pY685-VEC did not recognize VEC-Y685F mutant (left panels) but could bind to VEC-Y658F mutant (central and right panels) in pervanadate treated cells. Pixels presenting the co-localization of pY658- or pY685-VEC with total VEC are highlited in white. Scale bar: 50 μm. ( g ) Antibody pY658-VEC did not bind to immunoprecipitated VEC-Y658F mutant (central lanes), but recognized VEC-wt or VEC-Y685F mutant (left and right lanes). Conversely, antibody pY685-VEC did not recognize immunoprecipitated VEC-Y685F mutant (right lanes), but could bind to VEC-wt or VEC-Y658F mutant in pervanadate-treated cells (left and central lanes). ( h ) IP of wt hVEC followed by WB showed that antigen recognition by the commercially available antityrosine-phosphorylated-(Y658)-VEC antibody was increased upon pervanadate treatment. However, the antibody tested was also equally able to recognize the VEC-Δ622-702 mutant, in which the indicated tyrosine is not present. Data shown are representative of at least three independent experiments. 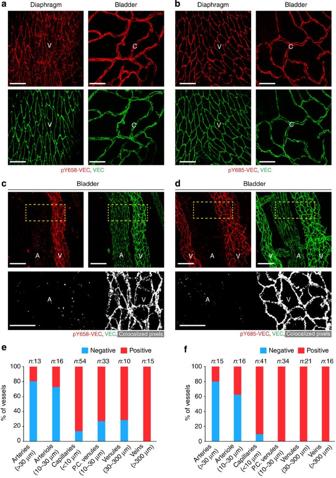Figure 2:In vivophosphorylation of VEC in veins but not in arteries. Staining of veins (V) and capillaries (C) of diaphragm and bladder with anti-pY658-VEC (a), anti-pY685-VEC (b) (both in red) and an antibody against total VEC (green). Both pYVEC antibodies label cell junctions. Scale bar: 50 μm. pY658-VEC (c) and pY685-VEC (d) antibodies stain endothelial junctions in veins but not in small arterioles (A). Scale bar: 50 μm. The boxes represent the area of magnification where pixels presenting VEC/pYVEC co-localization are highlighted in white. Scale bar: 20 μm. Data ina–dare representative of at least 10 independent mice per group. (e,f) Quantification of vessels positive or negative to either pY658-VEC (e) or pY685-VEC antibody (f); data are expressed as percentage of positive (red columns) and negative (blue columns) vessels grouped by diameter (μm),nis the total number of vessels considered for each group (P.C., postcapillaries). Full size image Figure 2: In vivo phosphorylation of VEC in veins but not in arteries. Staining of veins (V) and capillaries (C) of diaphragm and bladder with anti-pY658-VEC ( a ), anti-pY685-VEC ( b ) (both in red) and an antibody against total VEC (green). Both pYVEC antibodies label cell junctions. Scale bar: 50 μm. pY658-VEC ( c ) and pY685-VEC ( d ) antibodies stain endothelial junctions in veins but not in small arterioles (A). Scale bar: 50 μm. The boxes represent the area of magnification where pixels presenting VEC/pYVEC co-localization are highlighted in white. Scale bar: 20 μm. Data in a – d are representative of at least 10 independent mice per group. ( e , f ) Quantification of vessels positive or negative to either pY658-VEC ( e ) or pY685-VEC antibody ( f ); data are expressed as percentage of positive (red columns) and negative (blue columns) vessels grouped by diameter (μm), n is the total number of vessels considered for each group (P.C., postcapillaries). Full size image Constitutive VEC phosphorylation in veins In vivo staining of mice blood vessels with both pYVEC antibodies (pY658-VEC or pY685-VEC) and total VEC antibody revealed that pYVEC was detectable in endothelial cells of veins under resting conditions ( Fig. 2a ). The staining followed cell junctions in all endothelial cells along the whole length of the vessels. In striking contrast, endothelial cells of small arterioles were not stained by any of the pYVEC antibodies, but were stained by antibodies to total VEC ( Fig. 2c ). The different expression of pYVEC in veins and not in small arterioles was reproducible in all the tissues examined and clearly distinguished contiguous arterioles from veins ( Fig. 2c ). Quantification of pYVEC distribution in the different types of vessels is shown in Fig. 2e . As a control, we stained the vessels with antibodies directed to different junctional proteins (PECAM-1, β-catenin, p120) [22] . All antibodies stained the endothelial cell junctions of arteries and veins equally well ( Supplementary Fig. S1c,d ), demonstrating that the accessibility of the antibodies was comparable and that the general organization of junctions did not differ substantially in both the types of vessels. To test whether endothelial cells arterio/venous identity constitutively influences VEC phosphorylation, we examined freshly isolated venous and arterial endothelial cells in culture. We found that pYVEC staining in vitro did not differ in both the endothelial cell types ( Supplementary Fig. S1e ), suggesting that arterio/venous identity does not influence VEC phosphorylation per se but factors such as shear stress or hydrostatic pressure present in vivo may be important. Hemodynamic conditions modulate VEC phosphorylation We hypothesized that the observed difference in VEC phosphorylation in arteries and veins could be due to the hemodynamic conditions to which the endothelial cells are exposed. To test this hypothesis, cultured HUVEC were exposed to a range of different shear stresses ( Fig. 3a ). We found that in static conditions VEC phosphorylation was low, but was significantly increased by exposure to 3.5 dynes cm −2 , but then declined when shear stress was increased to up to 28 dynes cm −2 . At higher shears, VEC phosphorylation further decreased to baseline levels. 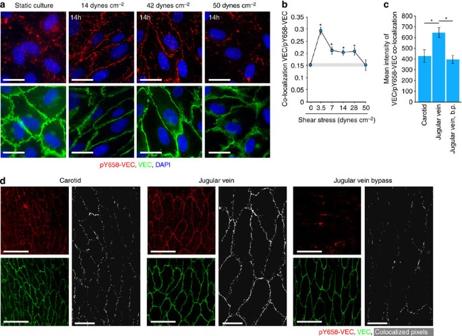Figure 3: Shear stress modulates VEC phosphorylation. (a,b) Parametric study of cultured HUVEC exposed to different levels of shear stress as indicated. Low and medium shear stress (from 3,5 dynes cm−2up to 28 dynes cm−2) increased pY658-VEC junctional staining as compared with static conditions. Further increase of shear stress up to 50 dynes cm−2(corresponding to high arterial flow) induced a progressive reduction of pY658-VEC junctional staining until levels similar to control cells. Scale bar: 20 μm. Chart in (b) shows the co-localization (VEC/pY658-VEC) data as Pearson’s correlation coefficient. Ten to 20 stacks were collected on different fields (each containing an average of 10 cells) for each sample under analysis. The grey area shows the co-localization value for static control plus/minus two times its s.e. Statistical comparisons of Pearson’s coefficients measured in different fields from two to three independent specimens were performed with non-parametric two-tailed Mann–Whitney tests (α=0.05); see Methods for details. (c) Mean fluorescence intensity of co-localized pY658-VEC and total VEC pixels as in (d). Statistical significance was determined on four individual animals by independent two-tailedt-test assuming unequal variances. (b.p., bypass,n=4 rat per group). (d) Untreated rat carotid artery showed lower pY658-VEC antibody staining as compared with the jugular vein. Exposure of jugular vein endothelium to arterial flow for 30 min significantly decreased pY658-VEC antibody staining. Scale bar: 50 μm. Pixels showing VEC/pY658-VEC co-localization (white) are highlighted in magnifications (scale bar: 20 μm). *P<0.01 by the above specified test. Figure 3: Shear stress modulates VEC phosphorylation. ( a , b ) Parametric study of cultured HUVEC exposed to different levels of shear stress as indicated. Low and medium shear stress (from 3,5 dynes cm −2 up to 28 dynes cm −2 ) increased pY658-VEC junctional staining as compared with static conditions. Further increase of shear stress up to 50 dynes cm −2 (corresponding to high arterial flow) induced a progressive reduction of pY658-VEC junctional staining until levels similar to control cells. Scale bar: 20 μm. Chart in ( b ) shows the co-localization (VEC/pY658-VEC) data as Pearson’s correlation coefficient. Ten to 20 stacks were collected on different fields (each containing an average of 10 cells) for each sample under analysis. The grey area shows the co-localization value for static control plus/minus two times its s.e. Statistical comparisons of Pearson’s coefficients measured in different fields from two to three independent specimens were performed with non-parametric two-tailed Mann–Whitney tests (α=0.05); see Methods for details. ( c ) Mean fluorescence intensity of co-localized pY658-VEC and total VEC pixels as in ( d ). Statistical significance was determined on four individual animals by independent two-tailed t -test assuming unequal variances. (b.p., bypass, n =4 rat per group). ( d ) Untreated rat carotid artery showed lower pY658-VEC antibody staining as compared with the jugular vein. Exposure of jugular vein endothelium to arterial flow for 30 min significantly decreased pY658-VEC antibody staining. Scale bar: 50 μm. Pixels showing VEC/pY658-VEC co-localization (white) are highlighted in magnifications (scale bar: 20 μm). * P <0.01 by the above specified test. Full size image The shear stress values to which vessels are exposed in vivo are much debated and vary between veins and arteries. For the in vitro studies above we refer to Kroll et al. [23] , who reported that venous shear stress range 0.76–7.6 dynes cm −2 while arterioles range 19–60.8 dynes cm −2 . To extend the study to in vivo conditions we switched to an experimental system in the rat, taking advantage of species cross-reactivity of antibody pY658-VEC. Figures 3c shows that VEC was phosphorylated in the jugular vein and, to a much lower extent, in the carotid artery. To expose venous endothelial cells to a higher shear stress we connected the carotid artery to the jugular vein to produce an in vivo shunt. Under these conditions pYVEC staining of venous endothelial cells was decreased. Overall, these observations show that VEC phosphorylation is influenced by hemodynamic conditions and suggest that at high shear rates phosphorylation of VEC tends to decrease. Src activation is required for shear-induced pYVEC Previous work showed that Src is implicated in VEC phosphorylation [11] . We investigated whether differences in activation of Src may explain the different phosphorylation of VEC in arteries and veins. In vivo staining with antibodies directed against Src or its active form, pY418-Src, showed that this kinase is localized at endothelial cell contacts both in arteries and in veins ( Fig. 4a , left panels). However, junctional Src is activated only in veins and not in arteries ( Fig. 4a , right panels). Accordingly, specific inhibitors of Src activation ( Fig. 4b ) inhibited pYVEC staining in vivo in veins ( Fig. 4d ), or in vitro in endothelial cells exposed to flow ( Fig. 4f ). These findings support the concept that hemodynamic conditions influence Src activation and, as a consequence, VEC phosphorylation in veins. 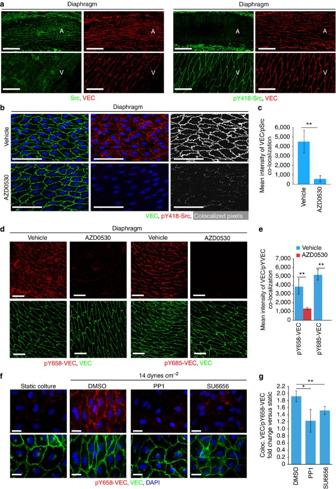Figure 4: Shear stress induced VEC phosphorylation is mediated by Src activation. (a) Src (green) and VEC (red) staining of arterial and venous endothelium in the mouse diaphragm. Staining presented in left panels shows junctional distribution of total Src in both vessel types (n=4 mice). Conversely, active Src (pY418-Src, right panels) is present at cell-to-cell contacts in veins only (n=4 mice). (b,c)In vivostaining for active Src (pY418-Src) of venous endothelium (mouse diaphragm) was abolished by treatment with a Src inhibitor (AZD0530). Mean fluorescence intensity of co-localized VEC and pY418-Src pixels is shown in (c). Data are mean±s.e.m. of five mice analysed. Statistical significance was determined by independent two-tailt-test assuming unequal variances. Scale bar: 50 μm. (d,e) VEC phosphorylation (pY658- or pY685-VEC in red, total VEC in green) of venous endothelium of mouse diaphragm was abrogated by AZD0530. Quantification in (e) reports mean fluorescence intensity of co-localized VEC/pY658-VEC (left) or pY685-VEC (right) pixels. Data are mean±s.e.m. of at least 10 veins analysed. Statistical significance was determined by independent two-tailt-test assuming unequal variances. Scale bar: 50 μm. (f,g) Flow-induced Y658-VEC phosphorylation in cultured HUVEC was abolished upon treatment with Src inhibitors PP1 or SU6656 by immunofluorescence (f). Co-localization (VEC/pY658-VEC) analysis (g) is reported as fold change versus static conditions. Statistical comparisons of Pearson’s coefficients measured in different fields from two to three independent specimens were performed with non-parametric two-tailed Mann–Whitney tests (α=0.05); see Methods for details. Scale bar: 20 μm. *P<0.05 and **P<0.01 by the above specified test. Figure 4: Shear stress induced VEC phosphorylation is mediated by Src activation. ( a ) Src (green) and VEC (red) staining of arterial and venous endothelium in the mouse diaphragm. Staining presented in left panels shows junctional distribution of total Src in both vessel types ( n =4 mice). Conversely, active Src (pY418-Src, right panels) is present at cell-to-cell contacts in veins only ( n =4 mice). ( b , c ) In vivo staining for active Src (pY418-Src) of venous endothelium (mouse diaphragm) was abolished by treatment with a Src inhibitor (AZD0530). Mean fluorescence intensity of co-localized VEC and pY418-Src pixels is shown in ( c ). Data are mean±s.e.m. of five mice analysed. Statistical significance was determined by independent two-tail t -test assuming unequal variances. Scale bar: 50 μm. ( d , e ) VEC phosphorylation (pY658- or pY685-VEC in red, total VEC in green) of venous endothelium of mouse diaphragm was abrogated by AZD0530. Quantification in ( e ) reports mean fluorescence intensity of co-localized VEC/pY658-VEC (left) or pY685-VEC (right) pixels. Data are mean±s.e.m. of at least 10 veins analysed. Statistical significance was determined by independent two-tail t -test assuming unequal variances. Scale bar: 50 μm. ( f , g ) Flow-induced Y658-VEC phosphorylation in cultured HUVEC was abolished upon treatment with Src inhibitors PP1 or SU6656 by immunofluorescence ( f ). Co-localization (VEC/pY658-VEC) analysis ( g ) is reported as fold change versus static conditions. Statistical comparisons of Pearson’s coefficients measured in different fields from two to three independent specimens were performed with non-parametric two-tailed Mann–Whitney tests (α=0.05); see Methods for details. Scale bar: 20 μm. * P <0.05 and ** P <0.01 by the above specified test. Full size image Detection of pYVEC is decreased by inflammatory mediators Next, we asked what the functional meaning of the distinct phosphorylation pattern of VEC in veins and arteries might be. We reasoned that the expression of pYVEC might increase the sensitivity of vessels to permeability-inducing agents. To test this possibility we treated mice with bradykinin, a well-documented permeability-increasing inflammatory mediator [24] , [25] , [26] . Four min after bradykinin injection we found a significant increase in permeability in veins, but not in arterioles, as detected by extravasation of fluorescent microspheres [24] ( Fig. 5a and Supplementary Fig. S2a ). The effect of bradykinin was fast, potent and reversible [24] , [25] . Surprisingly, in areas of increased permeability we noticed a strong decrease in pYVEC staining ( Fig. 5a ; Supplementary Fig. S2a ) that was restored within 10 min when also the baseline level of permeability was restored. A close analysis of endothelial junctions showed that pYVEC staining was decreased only in the areas of increased beads extravastion ( Fig. 5b ). Small gaps at cell-to-cell junctions can be observed (arrows) as described [24] , although only minor changes in total VEC staining at cell junctions was observed ( Fig. 5b , middle panels) suggesting that pYVEC represents a fraction of total VEC and is a specific target of bradykinin. In contrast, we did not detect extravasation of microspheres or change in VEC phosphorylation in arterioles ( Fig. 5a , asterisk). 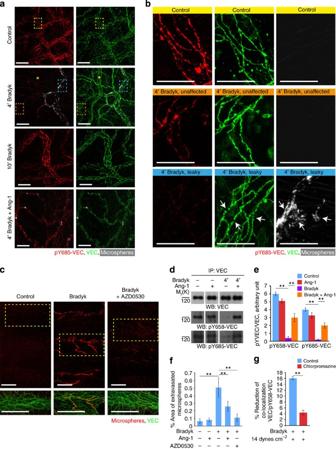Figure 5: pYVEC staining is decreased by bradykinin treatment. (a) At 4 min, bradykinin (bradyk) treatmentin vivostrongly increased venous permeability of the trachea vasculature, as measured by fluorescent microsphere extravasation (white), and markedly reduced pY685-VEC staining (red), VEC is shown in green. At 10 min permeability and pY685-VEC staining were restored. Permeability did not increase in small arteries (asterisk). Treatment with angiopoietin-1 (Ang-1) strongly inhibited the effect of bradykinin on both pY685-VEC staining and permeability. (b) Magnifications of the boxed areas for control and bradykinin-treated mice (4 min). Junctional pY685-VEC was strongly reduced in the sites of altered permeability while total VEC was still present with similar intensity than in control mice (lower panels and arrows). Middle panels show that in the areas unaffected by bradykinin treatment, pY685-VEC was only minimally altered. Staining with pY658-VEC antibody resulted in superimposable results (seeSupplementary Fig. S2a). Scale bars: 50 μm (left images) and 20 μm in magnified fields. (c) Bradykinin-induced vascular permeability in the mouse trachea was blocked by Src inhibitor AZD0530 as shown by extravasated microspheres (red, upper panels). Higher magnifications are shown in the lower panels and show VEC staining (green) and extravasated microspheres (red). Scale bar: 500 μm. (d) Immunoprecipitation (IP) of VEC from lung extracts showed that in the presence of bradykinin, phosphorylation of both Y658 and Y685 was reduced and Ang-1 prevented this effect. (e) Quantification of normalized band intensity as in (d). Data are mean±s.e.m. of five separate experiments. (f) Quantification of the areas covered by extravasated beads as in (a) and (c). Data are mean±s.e.m. of at least three mice considering 10 separate fields per mice in each group. Statistical significance was determined by analysis of variance test (e) or by independent two-tailedt-test assuming unequal variances (f). (g) Bradykinin reduces the co-localization of VEC with pY658-VEC in flow conditioned HUVEC (seeFig. 3a) while chlorpromazine inhibits this effect. Statistical comparisons were performed as inFig. 3b. *P<0.05 and **P<0.01 by the above specified test. Figure 5: pYVEC staining is decreased by bradykinin treatment. ( a ) At 4 min, bradykinin (bradyk) treatment in vivo strongly increased venous permeability of the trachea vasculature, as measured by fluorescent microsphere extravasation (white), and markedly reduced pY685-VEC staining (red), VEC is shown in green. At 10 min permeability and pY685-VEC staining were restored. Permeability did not increase in small arteries (asterisk). Treatment with angiopoietin-1 (Ang-1) strongly inhibited the effect of bradykinin on both pY685-VEC staining and permeability. ( b ) Magnifications of the boxed areas for control and bradykinin-treated mice (4 min). Junctional pY685-VEC was strongly reduced in the sites of altered permeability while total VEC was still present with similar intensity than in control mice (lower panels and arrows). Middle panels show that in the areas unaffected by bradykinin treatment, pY685-VEC was only minimally altered. Staining with pY658-VEC antibody resulted in superimposable results (see Supplementary Fig. S2a ). Scale bars: 50 μm (left images) and 20 μm in magnified fields. ( c ) Bradykinin-induced vascular permeability in the mouse trachea was blocked by Src inhibitor AZD0530 as shown by extravasated microspheres (red, upper panels). Higher magnifications are shown in the lower panels and show VEC staining (green) and extravasated microspheres (red). Scale bar: 500 μm. ( d ) Immunoprecipitation (IP) of VEC from lung extracts showed that in the presence of bradykinin, phosphorylation of both Y658 and Y685 was reduced and Ang-1 prevented this effect. ( e ) Quantification of normalized band intensity as in ( d ). Data are mean±s.e.m. of five separate experiments. ( f ) Quantification of the areas covered by extravasated beads as in ( a ) and ( c ). Data are mean±s.e.m. of at least three mice considering 10 separate fields per mice in each group. Statistical significance was determined by analysis of variance test ( e ) or by independent two-tailed t -test assuming unequal variances ( f ). ( g ) Bradykinin reduces the co-localization of VEC with pY658-VEC in flow conditioned HUVEC (see Fig. 3a ) while chlorpromazine inhibits this effect. Statistical comparisons were performed as in Fig. 3b . * P <0.05 and ** P <0.01 by the above specified test. Full size image We also treated mice with another permeability-increasing agent. Histamine acted in a way similar to bradykinin by reducing VEC phosphorylation in the areas of increased permeability ( Supplementary Fig. S2b,c ). Consistent with the staining, immunoprecipitation and western blot of lung extracts showed that bradykinin induced a significant decrease in pYVEC, as detected by both pY658-VEC and pY685-VEC antibodies ( Fig. 5d ). We also found that Src activation is required for bradykinin-induced permeability as pretreatment of mice with the Src inhibitor AZD0530 (see Fig. 4b ) inhibited the increase in permeability ( Fig. 5c ). As a further control, before bradykinin administration, we treated the mice with angiopoietin-1, which is known to stabilize the vasculature and counteract the action of several inflammatory mediators [9] , [24] , [25] , [27] , [28] , [29] . Angiopoietin-1 administration strongly reduced the effect of bradykinin on vascular permeability and counteracted the decrease in pYVEC-staining at junctions ( Fig. 5a ; Supplementary Fig. S2a ). A possible explanation of the strong reduction of VEC phosphorylation is the activation of some specific phosphatase. To test this possibility, we performed proteomic analysis (gel separation of proteins, in-gel digestion and LC-MS/MS analysis [30] ) of VEC-associated proteins in lung extracts after bradykinin stimulation of mice (10 mg kg −1 , for 3 min), but we could not detect associated phosphatases including VE-PTP, SHP2 or Dep-1, which are able to associate to VEC complex [17] , [31] (data not shown). Treatment of endothelial cells with siRNA targeting VE-PTP and Dep-1 increased resting VEC phosphorylation, as expected ( Fig. 6a and Supplementary Fig. S3e ). However, after activation with bradykinin, pYVEC at the membrane was reduced both in controls and in Dep-1 or VE-PTP siRNA-treated cells, indicating that inactivation of these phosphatases does not prevent the decrease of pYVEC after bradykinin treatment. 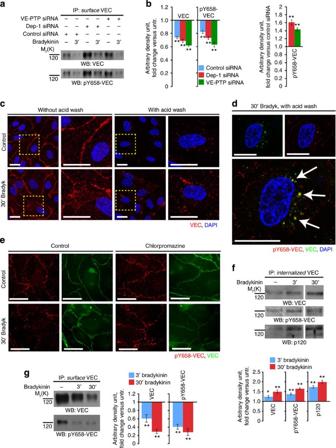Figure 6: Phosphorylated VEC is internalized. (a) Immunoprecipitation (IP) of surface VEC in HUVEC. Bradykinin treatment reduces surface VEC and its pY658 phosphorylated form. Treatment of the cells with siRNA targeting VE-PTP and Dep-1 increased resting VEC phosphorylation, but did not inhibit the decrease of surface amount of total and pYVEC induced by bradykinin. Western blot (WB) analysis of silencing efficiency (>70%) is shown inSupplementary Fig. S3e. (b) Quantification of surface VEC (left) and pY658-VEC (right) reduction in siRNA-treated cells (Control, Dep-1 or VE-PTP siRNA in blue, red or green, respectively) after bradykinin stimulus, fold change versus unstimulated cells. Right graph depicts the quantification (fold change versus control siRNA) of surface pY658-VEC in siRNA-treated cells (Dep-1 or VE-PTP siRNA in red or green, respectively). (c) 30 min bradykinin (bradyk) treatment of HUVEC, in the presence of chloroquine. Acid wash highlights the signal from internalized VEC (right panels and magnification). VEC internalization corresponded to partial disruption of endothelial junctions as can be observed in the absence of acid wash (left panels and magnification). Scale bars: 20 and 50 μm in magnifications. (d) Co-staining of VEC and pY658-VEC upon cell treatment with bradykinin and acid wash in the presence of chloroquine. Channels merge (bottom panel) shows that a fraction of internalized VEC is phosphorylated (arrows). Scale bars: 20 μm and 50 μm in magnified fields. (e) HUVEC showed a discontinuous junctional staining with pY658-VEC (in red), which was lost upon bradykinin treatment. This effect was prevented by chlorpromazine, a general inhibitor of endocytosis. VEC is shown in green. Scale bar: 50 μm. (f) IP of internalized VEC in HUVEC after 3 or 30 min bradykinin treatment. Internalized VEC was tyrosine (Y658) phosphorylated and still bound to p120. Quantification of normalized band intensities is shown in bottom panel. (g) IP of surface VEC. Bradykinin decreased the amount of total and pYVEC present on the surface. Quantification of normalized band intensities is shown in right panel. Data in (c,dande) are representative of at least three independent experiments per group. Data in (b), (f, bottom panel) and (g, right panel) are mean±s.e.m. of three independent experiments. *P<0.05 and **P<0.01 by independent two-tailedt-test assuming unequal variances. Figure 6: Phosphorylated VEC is internalized. ( a ) Immunoprecipitation (IP) of surface VEC in HUVEC. Bradykinin treatment reduces surface VEC and its pY658 phosphorylated form. Treatment of the cells with siRNA targeting VE-PTP and Dep-1 increased resting VEC phosphorylation, but did not inhibit the decrease of surface amount of total and pYVEC induced by bradykinin. Western blot (WB) analysis of silencing efficiency (>70%) is shown in Supplementary Fig. S3e . ( b ) Quantification of surface VEC (left) and pY658-VEC (right) reduction in siRNA-treated cells (Control, Dep-1 or VE-PTP siRNA in blue, red or green, respectively) after bradykinin stimulus, fold change versus unstimulated cells. Right graph depicts the quantification (fold change versus control siRNA) of surface pY658-VEC in siRNA-treated cells (Dep-1 or VE-PTP siRNA in red or green, respectively). ( c ) 30 min bradykinin (bradyk) treatment of HUVEC, in the presence of chloroquine. Acid wash highlights the signal from internalized VEC (right panels and magnification). VEC internalization corresponded to partial disruption of endothelial junctions as can be observed in the absence of acid wash (left panels and magnification). Scale bars: 20 and 50 μm in magnifications. ( d ) Co-staining of VEC and pY658-VEC upon cell treatment with bradykinin and acid wash in the presence of chloroquine. Channels merge (bottom panel) shows that a fraction of internalized VEC is phosphorylated (arrows). Scale bars: 20 μm and 50 μm in magnified fields. ( e ) HUVEC showed a discontinuous junctional staining with pY658-VEC (in red), which was lost upon bradykinin treatment. This effect was prevented by chlorpromazine, a general inhibitor of endocytosis. VEC is shown in green. Scale bar: 50 μm. ( f ) IP of internalized VEC in HUVEC after 3 or 30 min bradykinin treatment. Internalized VEC was tyrosine (Y658) phosphorylated and still bound to p120. Quantification of normalized band intensities is shown in bottom panel. ( g ) IP of surface VEC. Bradykinin decreased the amount of total and pYVEC present on the surface. Quantification of normalized band intensities is shown in right panel. Data in ( c , d and e ) are representative of at least three independent experiments per group. Data in ( b ), ( f , bottom panel) and ( g , right panel) are mean±s.e.m. of three independent experiments. * P <0.05 and ** P <0.01 by independent two-tailed t -test assuming unequal variances. Full size image pYVEC is internalized upon bradykinin treatment We hypothesized that pYVEC disappearance from junctions is due to endocytosis followed by degradation. To study this possibility, unfixed cells were incubated with anti-VEC antibodies and then activated by bradykinin in the presence of chloroquine, an inhibitor of protein degradation in lysosomes and recycling to the membrane [32] , [33] . Upon acid wash, antibodies linked to membrane-bound VEC were lost, while antibodies bound to internalized VEC could still be detected [33] . Bradykinin treatment strongly increased VEC internalization ( Fig. 6c ). Co-staining of internalized VEC with antibody pY658-VEC showed that a significant amount of internalized VEC was phosphorylated in tyrosine ( Fig. 6d ). Furthermore, by immunofluorescence analysis, bradykinin reduced pYVEC staining at junctions ( Fig. 6e ) and this effect was counteracted by chlorpromazine, an inhibitor of clathrin-dependent endocytosis [30] , [34] ( Fig. 6e ). Consistently, selective immunoprecipitation of internalized or surface VEC ( Fig. 6f ) upon bradykinin stimulation showed that surface pYVEC is reduced while internalized pYVEC is increased. These effects were detectable at 3 min and further increased at 30 min. The lasting presence of internalized VEC upon bradykinin stimulation in vitro, as compared with in vivo conditions, is likely due to the fact that cells were treated with chloroquine preventing protein degradation in intracellular vesicles. Consistently, flow-induced pY658-VEC co-localization with VEC was also significantly reduced by 3 min bradykinin treatment and this effect was abrogated by pretreatment of the cells with chlorpromazine ( Fig. 5g ). Thus, bradykinin induces internalization of pYVEC consistently with pYVEC disappearance from endothelial cell junctions in vivo . To test whether phosphorylation is required for bradykinin-induced VEC internalization, we analysed VEC-null endothelial cells reconstituted with VEC-wt or point mutants (VEC-Y658F and VEC-Y685F) unable to undergo phosphorylation in these specific tyrosine residues. We found that only VEC-wt could be internalized upon bradykinin treatment while both VEC-Y658F and VEC-Y685F were rather insensitive to this agent and remained on the cell surface ( Fig. 7a ). Furthermore, when cells were treated with Src inhibitor AZD0530, which inhibits VEC phosphorylation, bradykinin-induced internalization of the protein was inhibited ( Fig. 7c ). 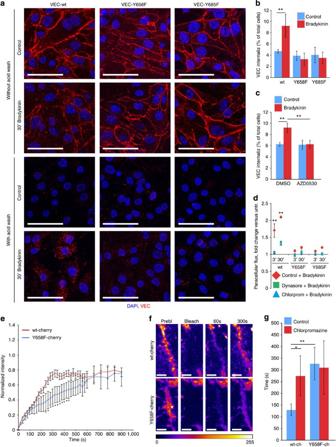Figure 7: VEC phosphorylation is necessary for its internalization. (a) VEC null murine endothelial cells were transduced with VEC-wt or non-phosphorylatable mutants (VEC-Y658F and VEC-Y685F). Treatment of the cells with 30 min bradykinin, in the presence of chloroquine, increased the number of cells showing internalized VEC-wt, but was ineffective on non-phosphorylatable mutants (lower panels, with acid wash). As observed for HUVEC, VEC internalization corresponded to partial disruption of endothelial junctions on cells expressing wt, but not mutant, VEC (upper panels, without acid wash). Scale bar: 50 μm. (b) Quantification of VEC internalization is reported as percentage of cells showing internalized VEC as in (a). Data are mean±s.e.m. of at least 100 cells analysed. (c) AZD0530 prevented bradykinin-induced VEC internalization. Data are shown as percentage of cells showing internalized VEC and are mean±s.e.m. of at least 100 cells analysed. (d) Three or 30 min bradykinin treatment increased paracellular permeability of cells expressing VEC-wt and, to a much lower extent, of cells expressing VEC-Y658F and VEC-Y685F (red diamonds, fold change over untreated cells). Dynasore (green squares) or chlorpromazine (blue triangles) were able to block the effect on cell permeability induced by bradykinin. Data are mean±s.d. of five replicates from a typical experiment out of three experiments performed. (e–g) FRAP experiment in HUVEC expressing fluorescent Y658F-cherry or wt-VEC-cherry revealed a reduced protein motility of Y658F-cherry mutant compared with wt-VEC-cherry. The strongest difference was at 300 s after bleach as shown in (f). Half-time of recovery (τ1/2) of wt-VEC-cherry protein was two fold higher upon chlorpromazine treatment (g). Y658F-cherry mutant presented a 2.5-fold higher basalτ1/2 than wt-VEC-cherry, and it was insensitive to chlorpromazine. Statistical significance was determined on at least 10 replicates. Scale bar is 4 μm. *P<0.05 and **P<0.01, by analysis of variance test (c,d) or by independent two-tailedt-test assuming unequal variances (b,eandg). Figure 7: VEC phosphorylation is necessary for its internalization. ( a ) VEC null murine endothelial cells were transduced with VEC-wt or non-phosphorylatable mutants (VEC-Y658F and VEC-Y685F). Treatment of the cells with 30 min bradykinin, in the presence of chloroquine, increased the number of cells showing internalized VEC-wt, but was ineffective on non-phosphorylatable mutants (lower panels, with acid wash). As observed for HUVEC, VEC internalization corresponded to partial disruption of endothelial junctions on cells expressing wt, but not mutant, VEC (upper panels, without acid wash). Scale bar: 50 μm. ( b ) Quantification of VEC internalization is reported as percentage of cells showing internalized VEC as in ( a ). Data are mean±s.e.m. of at least 100 cells analysed. ( c ) AZD0530 prevented bradykinin-induced VEC internalization. Data are shown as percentage of cells showing internalized VEC and are mean±s.e.m. of at least 100 cells analysed. ( d ) Three or 30 min bradykinin treatment increased paracellular permeability of cells expressing VEC-wt and, to a much lower extent, of cells expressing VEC-Y658F and VEC-Y685F (red diamonds, fold change over untreated cells). Dynasore (green squares) or chlorpromazine (blue triangles) were able to block the effect on cell permeability induced by bradykinin. Data are mean±s.d. of five replicates from a typical experiment out of three experiments performed. ( e – g ) FRAP experiment in HUVEC expressing fluorescent Y658F-cherry or wt-VEC-cherry revealed a reduced protein motility of Y658F-cherry mutant compared with wt-VEC-cherry. The strongest difference was at 300 s after bleach as shown in ( f ). Half-time of recovery ( τ 1/2) of wt-VEC-cherry protein was two fold higher upon chlorpromazine treatment ( g ). Y658F-cherry mutant presented a 2.5-fold higher basal τ 1/2 than wt-VEC-cherry, and it was insensitive to chlorpromazine. Statistical significance was determined on at least 10 replicates. Scale bar is 4 μm. * P <0.05 and ** P <0.01, by analysis of variance test ( c , d ) or by independent two-tailed t -test assuming unequal variances ( b , e and g ). Full size image The effect of bradykinin on endothelial permeability in vitro was strongly reduced in VEC mutant cells ( Fig. 7d ). Moreover, pretreatment of cells expressing VEC-wt with two inhibitors of protein internalization (chlorpromazine or dynasore) reduced bradykinin-induced permeability to the same level observed in cells expressing Y658F or Y685F mutants ( Fig. 7d ). Finally, to test whether VEC protein displays a higher mobility on the cell membrane when it is phosphorylated on Y658, we performed fluorescence recovery after photobleaching (FRAP) [35] , [36] analysis of VEC recovery at cell-to-cell junctions using Cherry-conjugated wild-type or Y658F mutant ( Fig. 7e–g ). In previous work it was found that the recovery at junctions of E-cadherin after photobleaching is due to endocytosis and subsequent exocytosis [35] . We observed that membrane recycling of VEC-Y658F was significantly slower than VEC-wt ( Fig. 7e ). Chlorpromazine increased the halftime of recovery of VEC-wt but not of Y658F mutant, suggesting that the constitutive mobility of the protein is mediated by its internalization and that Y658 phosphorylation has a central role in this part of the process. VEC is ubiquitinated after bradykinin treatment In search for a mechanism of pYVEC internalization and degradation we tested whether ubiquitin was involved in these processes. We found that bradykinin treatment induced VEC ubiquitination in vivo ( Fig. 8a ) and in vitro ( Fig. 8b ). Importantly, VEC ubiquitination in vivo correlated with the decrease in pYVEC detection ( Fig. 8a ) and staining (see Fig. 5a ). Furthermore, Y658F and Y685F point mutants showed poor, if any, ubiquitination after bradykinin treatment ( Fig. 8c ) supporting the concept that VEC phosphorylation in these tyrosines is required for its ubiquitination. These data also suggest that ubiquitination is involved in pYVEC internalization and disappearance from junctions in vivo . 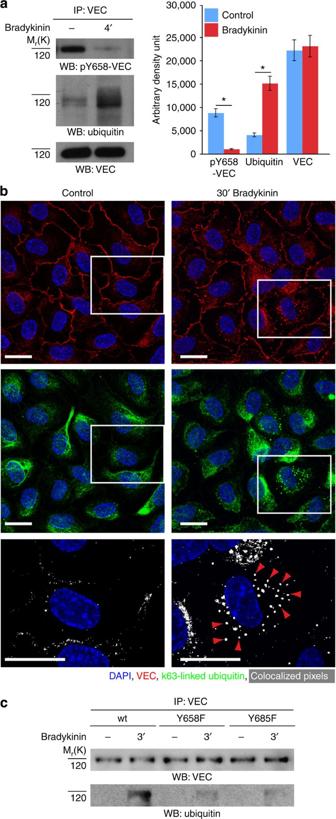Figure 8: Bradykinin induced VEC internalization is coupled by ubiquitination. (a) IP of lung extracts followed by WB revealed that, at 4 min after bradykinin, reduction of VEC recognition by pY-VEC antibodies was accompanied by a strong increase in ubiquitination. Quantification of band intensity is shown as absolute values on the right panel. (b) HUVEC were treated, in presence of chloroquine, with bradykinin or left untreated. Bradykinin-induced VEC internalization (red staining) and co-localization in intracellular vesicles with K63-linked ubiquitin (green staining) in HUVEC cells. Pixels presenting VEC and ubiquitin colocalization are highlighted in white in the magnified fields (bottom). Red arrowheads point to internalized VEC. Data are representative of at least three independent experiments. Scale bar: 20 μm. (c) IP of wt or point mutated VEC followed by WB for ubiquitin showed that bradykinin induces stronger ubiquitination of wt protein than of Y658F- or Y685F-VEC mutants. Data in (a) are mean±s.e.m. of three independent experiments. *P<0.01 by independent two-tailedt-test assuming unequal variances. Figure 8: Bradykinin induced VEC internalization is coupled by ubiquitination. ( a ) IP of lung extracts followed by WB revealed that, at 4 min after bradykinin, reduction of VEC recognition by pY-VEC antibodies was accompanied by a strong increase in ubiquitination. Quantification of band intensity is shown as absolute values on the right panel. ( b ) HUVEC were treated, in presence of chloroquine, with bradykinin or left untreated. Bradykinin-induced VEC internalization (red staining) and co-localization in intracellular vesicles with K63-linked ubiquitin (green staining) in HUVEC cells. Pixels presenting VEC and ubiquitin colocalization are highlighted in white in the magnified fields (bottom). Red arrowheads point to internalized VEC. Data are representative of at least three independent experiments. Scale bar: 20 μm. ( c ) IP of wt or point mutated VEC followed by WB for ubiquitin showed that bradykinin induces stronger ubiquitination of wt protein than of Y658F- or Y685F-VEC mutants. Data in ( a ) are mean±s.e.m. of three independent experiments. * P <0.01 by independent two-tailed t -test assuming unequal variances. Full size image Cadherin internalization and degradation may be also regulated by p120(refs 18 , 19 , 33 , 37 , 38 ) and VEC phosphorylation in Y658 may reduce the affinity for p120 binding, promoting its internalization [18] , [39] . We found that bradykinin does not induce p120 dissociation from VEC as shown by co-immunoprecipitation assay of total and internalized VEC ( Supplementary Fig. S3c and Fig. 6f respectively), or by codistribution of internalized VEC and p120 ( Supplementary Fig. S3a, b ). Moreover, in vivo p120 codistributed with pY-VEC at endothelial junctions ( Supplementary Fig. S1d ). Thus, under our experimental conditions, we have been unable to demonstrate a clear link between p120 dissociation and VEC internalization. VEC has a central role in the control of vascular permeability, and deregulation of its expression or function is associated with increased oedema and vascular fragility [1] , [2] , [3] , [7] , [8] , [40] . While recent studies have begun to uncover the mechanisms through which VEC activity is regulated in vitro [7] , [9] , [17] , [41] , [42] , [43] , few data [11] , [31] , [44] , [45] are available on VEC functional modulation in vivo . In starved endothelial cells in vitro, VEC phosphorylation in tyrosine is extremely low but is increased by permeability-increasing agents such as vascular endothelial growth factor (VEGF) or leucocyte adhesion [14] , [41] , [43] . By in vivo staining we observed that VEC is phosphorylated in Y658 and Y685 in veins also in the absence of inflammatory agents or vascular leakage. Therefore, VEC phosphorylation at these two tyrosine residues in vivo is not sufficient per se to reduce endothelial barrier function. Nevertheless, as discussed below, VEC phosphorylation may act as a priming mechanism to sensitize veins to permeability-inducing agents. An important question is how VEC phosphorylation is modulated in vivo . We report evidence that hemodynamic conditions modulate VEC phosphorylation through Src activity and that this mechanism acts mostly in veins but not in small arteries. We have shown that in veins there is a constitutive and prolonged activation of Src, which in turn may mediate VEC phosphorylation. Activation of Src family kinases and the subsequent VEC phosphorylation has been described as a critical step in the induction of permeability by growth factors and inflammatory cytokines [9] , [11] , [44] . In vivo we observed that Src is constitutively activated in veins and this is necessary but not sufficient to induce vascular leakage. These observations are in agreement with Adam et al. [46] who showed that phosphorylation of VEC by Src was not sufficient to decrease barrier function of cultured endothelial cells. The reasons why the above phenomena do not occur in arteries are not clear, notwithstanding the multiple differences that exist between arterial and venous vessels. These differences include the pattern and degree of investment by smooth muscle cells and/or pericytes, electrical coupling, distribution of endothelial markers such as ephrins and receptors to inflammatory mediators, and others [1] , [47] , [48] . The data reported here suggest that hemodynamic factors also may modulate Src activity and, as a consequence, VEC phosphorylation. As reported here VEC phosphorylation is influenced by shear stress in vitro and exposure of venous endothelial cells to arterial blood flow in vivo leads to a decrease in VEC phosphorylation. Although further work is required to define this mechanism in detail, data are in favour of a shear-sensing mechanism that modulates VEC phosphorylation. An interesting candidate is the endothelial mechanosensory complex formed by VEC, PECAM-1 and VEGFR-2. PECAM-1 has been shown to bind directly to Src and the binding is required for Src activation under shear [49] . We cannot, however, exclude that other hemodynamic factors such as hydrostatic pressure may contribute to low VEC phosphorylation in arteries. We also made efforts to understand the functional meaning of the constitutive VEC phosphorylation in vivo . As most inflammatory mediators act selectively and rapidly on veins, a tempting speculation is that VEC phosphorylation is a prerequisite for a rapid and fully reversible opening of endothelial junctions. As for other cadherins, VEC endocytosis reduces endothelial cells barrier function [2] , [9] , [37] , [38] , [50] . We found that bradykinin induces a quick disappearance of pY658 and pY685 VEC from junctions which, from the data collected in vitro , we interpret as internalization. When we used VEC point mutants Y658F and pY685F to inhibit phosphorylation we also blocked bradykinin-induced VEC internalization and increase in vascular permeability in vitro . It seems, therefore, that phosphorylation of VEC at these two tyrosine residues is required for bradykinin-induced vascular leakage. To further elucidate the pathway through which pYVEC contributes to its internalization and possibly degradation we considered that cell–cell contacts are sites for recruitment of the ubiquitination machinery [30] , [50] , [51] . Tyrosine phosphorylation of E-cadherin attracts Hakai, an E3 ubiquitin-ligase, which mediates its ubiquitination and endocytosis [50] . In agreement with this observation, we report here that activation by bradykinin leads to VEC ubiquitination and that this process requires tyrosine phosphorylation of Y658 and Y685. The decrease in phosphorylation of Y658 and Y685 in VEC may also be due to association to phosphatases. As above, the best candidates that were previously found to associate to VEC are VE-PTP [52] and Dep-1 (ref. 17 ). However, the knockdown of these phosphatases did not prevent the decrease in VEC phosphorylation upon bradykinin activation. Moreover, proteomic analysis of lung extracts of mice treated with bradykinin did not detect phosphatases associated to VEC complex. Thus, we have been unable to find, at least in our experimental system, a clear evidence for the role of phosphatases in regulating VEC phosphorylation. We did not perform a detailed analysis of the role of each tyrosine present in the cytoplasmic tail of VEC but focused on Y658 and Y685 instead. Both tyrosines are phosphorylated in venous endothelium, and in vitro studies on VEC phosphomimetic mutants show that Y658 phosphorylation is important in VEC internalization [18] , [39] . Phosphorylation of VEC at Y658 may reduce its association to p120 and induce its internalization [18] , [34] . Under the different experimental conditions used here, however, we have been unable to detect a significant dissociation of p120 from internalized pYVEC. Others [46] using endothelial cells transfected by a constitutive active src, which induced pY658 phosphorylation, could not observe detachment of p120. Our data are consistent with this last report. These observations do not exclude that p120 is important for the stability of VEC at the membrane. However, detachment of p120 is unlikely to be the only way through which cadherins are internalized. Gavard et al. [10] reported that VEGF-mediated VE cadherin phosphorylation in the highly conserved Ser-665 induces the recruitment of β-arrestin2, VEC internalization and increase in permeability in cultured cells. We do not know whether phospho Ser-665 also contributes to bradykinin-induced VEC internalization at this stage. However, we cannot exclude that VEC activation by permeability increasing agents may result in different steps of phosphorylation which, downstream, contribute to the internalization of the protein. Lambeng et al. [44] describe, in organ extracts, VEC tyrosine phosphorylation under both resting and hormone-activated conditions. Interestingly and consistently with our data, phosphorylation of VEC was observed also under resting conditions in some organs such as the lung. When angiogenesis was stimulated by treatment with hormones, total VEC phosphorylation increased but only in uterus and ovary. Using heart extracts, Weis et al. [11] show increased VEC phosphorylation after VEGF treatment and inhibition of such an effect by Src inhibitors. The stimuli and the organs studied are different from those considered in our paper. Furthermore, the use of organ extracts does not allow a detailed analysis of positive or negative vessels. It is conceivable that angiogenic stimuli increase tyrosine phosphorylation in the growing vasculature and as final result, cause an increase in tyrosine phosphorylation of the whole organ extract. In conclusion, the data presented here help to draw a picture of how VEC processing is regulated in vivo by inflammatory mediators such as bradykinin or histamine. We report that VEC may be phosphorylated in Y658 and Y685 in veins through the action of hemodynamic forces. Our data suggest that phosphorylation in these tyrosines sensitizes VEC to the action of bradykinin, which induces rapid pYVEC internalization and ubiquitination. pYVEC in veins may, therefore, be important to prime the protein into a dynamic state that promotes, upon activation, its rapid internalization, leading to the quick and reversible opening of endothelial cells junctions and plasma leakage. We speculate that any agent capable of inhibiting VEC phosphorylation may effectively reduce vascular permeability induced by inflammatory agents. Animals and in vivo treatments C57BL/6J wt (20–25 g) mice (Charles River) were used. Mice anaesthetized with Avertin (2,2,2-tribromoethanol, 500 mg kg −1 intraperitoneally) were injected intravenously with bradykinin (10 mg kg −1 , Sigma), histamine (50 μmol kg −1 , Sigma) or 0.9% NaCl for the indicated time. For immunofluorescence analysis, 1 min before fixation, blue or green fluorescent microspheres (0.1 μm diameter, 50 μl, Duke Scientific) were intravenously injected. COMP-ang-1 expressing adenovirus (10 9 plaque-forming units) [28] were injected via the tail vein. Age-matched control mice received an injection of adenovirus expressing GFP. Eight days later, mice were challenged by intravenous injection of bradykinin (as above). AZD0530 (kind gift of Astra Zeneca) or vehicle (following the manufacturer’s instructions) was orally administered (25 mg kg −1 , 6 h). For carotid-jugular bypass, rats were anaesthetized with pentobarbital (50 mg kg −1 intraperitoneally) and injected with heparin (1000 U kg −1 intraperitoneally) 30 min before surgery. A heparinized polyethylene catheter (PE-60; Intramedic, Becton Dickinson) was inserted into the left carotid artery on one side and into the right jugular vein on the other side. Arterial blood flow deviation, from carotid artery to jugular vein, was applied for 30 min. Antibodies The following antibodies were used: goat anti-VEC (1:200, Santa Cruz), rat anti-mouse-VEC (5 μg ml −1 , BV13 (ref. 53 ) or 1:500, BD Transduction Laboratories), mouse anti-human-VEC (10 μg ml −1 , BV6) [54] , mouse anti-p120 (1:100, BD Transduction Laboratories), rabbit anti-β-catenin (1:200, Abcam), hamster anti-CD31 (1:500, Chemicon), rabbit anti-p120 and rabbit anti-cSrc (1:200 and 1:100 Santa Cruz), rabbit anti-phospho-Tyr 418-Src (1:100, Invitrogen), mouse anti-ubiquitin P4D1 (1:1,000, Santa Cruz), rabbit anti-K63-linked-polyubiquitin clone Apu3 (1:250, Millipore), rabbit anti-VEC (pY658) (1:1,000, Biosource), goat anti-Dep-1 (1:200, PTPRJ) (R&D System), Vinculin (1:1,000, Sigma). Affinity purified rabbit antibody to VE-PTP (PTPRB, 5 μg ml −1 ), pY658-VEC and pY685-VEC were produced and purified by New England Peptide. Antibodies pY658-VEC and pY685-VEC (10 μg ml −1 ) in PBS containing 1% bovine serum albumin (BSA) were further purified by three incubation cycles on VEC null endothelial cells (30 min VEGF stimulated, fixed, permeabilized and blocked as described in the relative section) for 1 h at room temperature and used for immunofluorescence or western blot (1 or 5 μg ml −1 ). Peptide-competition was obtained by incubating the antibodies with a 200-fold molar excess of the relative phosphorylated or non-phosphorylated peptide for 45 min at room temperature. Secondary antibodies for immunofluorescence were donkey antibodies to the appropriate species conjugated with Alexa-Fluor 488, 555 or 647 (1:400, Molecular Probes). Cells and in vitro treatments HUVEC and murine endothelial cells genetically ablated for VEC (VEC-null) were obtained and cultured as described [55] . VEC null or HUVEC were lentiviral transduced to express mVEC (see ‘Constructs’). CHO cells were cultured and transfected to express mVEC-mutants (see ‘Constructs’) using standard techniques. To knock down human VEC, PTPRB (VE-PTP) or PTPRJ (Dep-1) in HUVEC we used ON-TARGET plus SMART pool siRNAs from Dharmacon and the corresponding Stealth siRNAs control. Transfection was performed with LipofectAMINE 2,000 (Invitrogen) following the manufacturer’s instructions. Arterial and venous cells were isolated as described [56] . Confluent HUVEC or murine endothelial cells were rendered quiescent for 3 or 24 h, respectively, in MCDB131 medium (Invitrogen) containing 1% BSA. Bradykinin (1 μM, for the indicated time), chloroquine (300 μM or 100 μM, 3 h), chlorpromazine (5 μg ml −1 , 30 min), sodium pervanadate (obtained by adding to the cells 0.2 mM sodium orthovanadate and 0.4 mM H 2 O 2 , 5 min), AZD0530 (1 μM, 3 h), Cycloheximide (0.1 mg ml −1 , 30 min), Dynasore (60 μM, 30 min) COMP-Ang-1 (200ng/ml) or VEGF (80 ng ml −1 , 10 min) was added at 37 °C. Constructs mVEC constructs (VEC-wt, VEC-Y658F, VEC-Y685F) were produced using standard molecular biology procedures. Mutated VEC cytoplasmic tails were amplified by PCR as two fragments carrying the mutations and the restriction sites necessary for sub-cloning. Wild-type cytoplasmic tail was then replaced with the mutated versions to generate full length mutated VEC complementary DNAs. mCherry complementary DNA was subcloned into the pEGFP-N2 (Clontech) in place of EGFP sequence. VEC (wt and Y658F mutant) were then subcloned to generate fusion proteins. VEC constructs were introduced in lentiviral plasmids to produce lentiviral vectors, as described [57] . Human VEC-Δ622-702 was described elsewhere [20] . Flow experiments A custom-built flow chamber consisting of two parallel plates made of polymethyl-methacrylate was used to apply uniform shear stress on HUVEC monolayers. While the lower plate was flat, a rectangular channel was engraved on the upper plate with an automatic milling machine. HUVEC were grown to confluence on a patch of copolymer 2-norbornene-ethylene [58] . The patch was then placed on the lower plate and the upper plate was mounted to form a sealed channel of parallel-plate geometry. The actual shear stress ( τ ) applied to the cells can be expressed in terms of volumetric flow rate ( Q ), medium viscosity ( μ , 8.4 × 10 −4 Pa·s) [59] , width ( w, 20 mm) and height ( h, 0.3 mm ) of the channel: τ =6 Qμ / wh 2 . In our setup, flow rates of 30, 90 or 107 ml min −1 were applied to obtain shear stress values of 3.5, 7, 14, 28, 42 or 50 dynes cm −2 , respectively. The indicated flow rates were controlled using a peristaltic roller pump (Model 66, Harvard Apparatus). Cells were fixed after 14 h of constant flow. PP1 (10 μM, Enzo Life Sciences) or dimethylsulphoxide was added to the culture media before the onset of flow. SU6656 (10 μM, Sigma) was added to the culture media 30 min before fixation. Chlorpromazine or chloroquine were added to the culture media 30 min or 3 h (respectively) before bradykinin treatment. Co-localization data originate from multichannel fluorescence stacks collected using a Nikon-Ti (Nikon, Japan) wide-field microscope implemented with an Orca R2 CCD camera (Hamamatsu, Japan) and a X60/1.2 NA water immersion objective (Nikon). For each stack a single value of the Pearson’s coefficient (ranging between−1 and 1) was measured imposing a threshold value (calculated based on the algorithms by Costes et al. , [60] ) for green and red channels using the ‘co-localization analysis’ section of Imaris (Bitplane). Fluorescence recovery after photobleaching HUVEC expressing mCherry-constructs were grown to confluence on μ-slide 8-well (Ibidi). Chlorpromazine and/or Cycloheximide were added to the media 30 min before FRAP experiment. FRAP was performed as specified in Supplementary Methods . Immunofluorescence Cells were fixed and permeabilized with 3% paraformaldehyde, 0.5% Triton X100 in PBS for 3 min followed by further 15 min fixation with 3% paraformaldehyde in PBS. After anaesthesia, mice vasculature was perfused as described [24] . Trachea, diaphragm, urinary bladder or 9.5 dpc embryos were immersed in 1% paraformaldehyde in 0.1% triethanolamine, pH 7.5, containing 0.1% Triton X100 and 0.1% NP-40 for 1 h at room temperature. For immunostaining of tissues or cells, primary or secondary antibodies were diluted in 5% BSA, 5% donkey serum in PBS. CCD camera on epifluorescence microscope (Leica) or Leica TCS SP2 confocal microscopy were used. ImageJ (NIH) was employed for data analysis. Figures were assembled using Adobe Photoshop and Adobe Illustrator. Only adjustments of brightness and contrast were used in the preparation of the figures. For comparison purposes, different sample images of the same antigen were acquired under constant acquisition settings. Immunoprecipitation and western blotting For additional detail see Supplementary Methods . Briefly, for internalized or surface VEC immunoprecipitations, antibody–antigen (BV6) binding was performed in living cells before or after (respectively) pharmacological treatment at 4 °C. After six washes with PBS (containing calcium and magnesium ions) to remove the unbound antibody, cells were treated as follows: for internalized VEC immunoprecipitation, cells were treated in complete medium at 37 °C. To remove cell surface bound antibody while retaining internalized antibody, cells were acid washed five times in PBS, pH 2.7, containing 25 mM glycine and 3% BSA before lysis in JS buffer (see Supplementary Methods ). For surface VEC immunoprecipitation, cells were lysed immediately in JS buffer. Mouse lungs were collected and homogenized in modified radioimmunoprecipitation assay buffer buffer (see Supplementary Methods ). Protein concentrations were determined using a BCA Protein Assay Kit (Pierce) following the manufacturer’s instructions. Internalization assay Internalization assays were performed as previously described [33] . Briefly, to measure internalization of endogenous VEC, confluent HUVEC (or murine endothelial cells) were treated with 300 μM (or 100 μM) chloroquine. BV6 (or BV13) antibody was incubated with cells at 4 °C for 1 h in MCDB131 with 1% BSA medium. Cells were rinsed in ice-cold MCDB131 to remove unbound antibody and then treated with 1 μM bradykinin. Cells were acid or neutral (as indicated) washed five times and processed for immunofluorescence. Gelatine–glutaraldehyde crosslinking To enhance endothelial cell adhesion, slides were coated with glutaraldehyde-crosslinked gelatin as described in Supplementary Methods . Paracellular flux tracer analysis Endothelial cells were seeded on 0.4 μm pore-size Transwell Permeable Supports (Corning), cultured in complete culture medium and assayed for permeability to fluorescein isothiocyanate-dextran (70 kDa) (Sigma,) as described [57] . Study approval Procedures involving animals and their care conformed to institutional guidelines in compliance with national (4D.L.N.116, G.U., supplement 40, 18-2-1992) and international (EEC Council Directive 86/609, OJL358,1,12-12-1987, National Institutes of Health’s Guide for the Care and Use of Laboratory Animals , and United States National Research Council 1996) law and policies. All efforts were made to minimize the number of animals used and their suffering. How to cite this article: Orsenigo, F. et al. Phosphorylation of VE-cadherin is modulated by hemodynamic forces and contributes to the regulation of vascular permeability in vivo . Nat. Commun. 3:1208 doi: 10.1038/ncomms2199 (2012).